Nanoparticle-templated nanofiltration membranes for ultrahigh performance desalination Nanofiltration (NF) membranes with ultrahigh permeance and high rejection are highly beneficial for efficient desalination and wastewater treatment. Improving water permeance while maintaining the high rejection of state-of-the-art thin film composite (TFC) NF membranes remains a great challenge. Herein, we report the fabrication of a TFC NF membrane with a crumpled polyamide (PA) layer via interfacial polymerization on a single-walled carbon nanotubes/polyether sulfone composite support loaded with nanoparticles as a sacrificial templating material, using metal-organic framework nanoparticles (ZIF-8) as an example. The nanoparticles, which can be removed by water dissolution after interfacial polymerization, facilitate the formation of a rough PA active layer with crumpled nanostructure. The NF membrane obtained thereby exhibits high permeance up to 53.5 l m −2 h −1 bar −1 with a rejection above 95% for Na 2 SO 4 , yielding an overall desalination performance superior to state-of-the-art NF membranes reported so far. Our work provides a simple avenue to fabricate advanced PA NF membranes with outstanding performance. Aggravated by rapid population and economic growth, water contamination and scarcity have evolved to be a global challenge [1] , [2] . Extensive research has been devoted to developing advanced materials [3] , [4] and technologies [5] to augment fresh water supply by either seawater/brackish desalination or wastewater reuse. Of all existing desalination technologies, pressure-driven membrane-based technologies, such as reverse osmosis (RO) and nanofiltration (NF), are the most energy-efficient and technologically mature. In particular, NF membrane rejects multivalent salts and organic molecules with molecular weight cut-off (MWCO) > 200 Da, [6] , [7] rendering NF an ideal water treatment technology for low-energy, high-throughput desalination applications in which ultra-high rejection of monovalent ions is not required. These applications include, but are not limited to, treating industrial process streams [8] , decontaminating wastewater [9] , and softening brackish groundwater [10] . State-of-the-art NF membranes are based on a thin film composite (TFC) design [11] , which deposits a polyamide (PA) active layer, formed by interfacial polymerization, on top of a porous support layer that is typically an ultrafiltration (UF) [12] or a microfiltration (MF) membrane [13] , [14] . Such a TFC structure yields high performance membranes with strong mechanical integrity, and enables cost-effective and scalable membrane manufacturing. Although significant improvement has been made over the past decades to improving the performance of TFC NF membrane, the current permeance of TFC NF membranes is still not high. Further enhancing the permeance while maintaining a high-solute rejection rate can significantly reduce the membrane area required to achieve a target water production rate, thereby reducing the capital cost of NF and rendering it more affordable. The performance of TFC NF membrane, in terms of permeance and selectivity, is primarily determined by the PA active layer that is responsible for solute rejection. The regulation and control of the molecular and structural characteristics of the PA layer are thus of great importance in improving the performance of TFC NF membranes. Extensive effort has been dedicated to enhance the permeance of this active layer without sacrificing its selectivity. One viable strategy is to tailor the intrinsic properties of the active layer through either designing the polymer structure at the molecular level [15] , [16] , [17] , [18] or incorporating hydrophilic nanomaterials into the layer [19] , [20] , [21] . The main rationale of this strategy is to reduce the resistance of water transport across the active layer and thereby improve permeance. However, significant change of water transport properties in the PA-based active layers is hard to achieve because water transport is heavily restricted by the highly cross-linked polymer chains in a tortuous manner [22] . Another strategy to achieve a high permeance is to make thinner active layers to reduce water transport resistance [23] , [24] , [25] , [26] . This may be achieved by controlling the interfacial polymerization process where amine monomers diffusing from the aqueous phase rapidly react with the acid chloride diffusing from the organic phase. However, precise control of the interfacial polymerization process is challenging as the interfacial reaction on conventional polymeric UF/MF membranes is diffusion limited. Therefore, the typical thickness of PA active layer ranges from tens to hundreds of nanometers. A possible strategy to obtain a thin PA active layer with controlled interfacial reaction is to introduce interlayer media, such as inorganic nanostrands film [27] , carbon nanotube network layer [28] , [29] , and cellulose nanocrystals film [30] , etc. on top of commercial polymeric UF/MF membrane as the support layer. These interlayer media provide more uniform substrate pores and optimized water wetting property than conventional polymeric UF/MF membranes, which in turn enable more homogeneous distribution of the monomer solutions and more effective control of monomer release in interfacial polymerization. Using this approach, thin PA active layers with thickness near 10 nm have been achieved successfully. The resulting membranes with ultrathin PA layers exhibited substantially higher permeance. While this strategy of reducing active layer is effective in enhancing membrane permeance, further improvement of membrane performance following this strategy is limited, as it will become extremely challenging to prepare defect-free active layers that are even thinner than the state-of-the-art. Undoubtedly, increasing the effective permeable area of ultrathin PA active layer is a preferred route on the premise of no other features losing. Here we report a novel strategy of designing a TFC NF membrane with an unprecedented permeance via a nanostructure-mediated interfacial polymerization process in which nanoparticles are preloaded as sacrificial templating materials on a support porous membrane. These preloaded nanoparticles create rough and irregular nanostructure on the surface of support membrane. Thus, the interfacial polymerization of piperazine and trimesoyl chloride occurs over such a rugged surface with nanoscale roughness. After polymerization, these nanoparticles can be readily removed by water dissolution, forming a thin PA active layer with extensive crumpled nanoscale structures. This crumpled structure significantly increases the available area for water permeation per projected area on the support. The resulting PA TFC membrane exhibits an unprecedentedly high permeance up to 53.2 l m −2 h −1 bar −1 while maintaining a high rejection of 95.2 % for Na 2 SO 4 . This is the most permeable TFC PA NF membrane with a satisfactory level of rejection (for NF applications), outperforming all existing NF membranes to the best of our knowledge. Fabrication of crumple nanofiltration membrane The key to achieve the crumpled active layer structure is to pre-load nanoparticles as a sacrificial template on the porous support membrane for interfacial polymerization. Here, polydopamine (PD) decorated MOF ZIF-8 nanoparticles (PD/ZIF-8) with controlled particle sizes of 30–400 nm are used as representative sacrificial templates, as schematically illustrated in Fig. 1a . In order to ensure homogeneous and well-controlled loading of PD/ZIF-8 nanoparticles, a composite membrane, prepared by depositing an ultrathin layer of single-walled carbon nanotube (SWCNTs) network onto a commercial polyether sulfone (PES) MF membrane, was used as the porous support. Then a typical interfacial polymerization process, in which diamine monomer piperazine (PIP) and trimesoyl chloride (TMC) reacts at water–hexane interface to form the PA selective layer, was induced on the surface of such a support loaded with PD/ZIF-8 nanoparticles. Upon the completion of the polymerization reaction, the as-prepared NF composite membrane was immersed into water to dissolve the PD/ZIF-8 nanoparticles. A TFC PA NF membrane with crumpled structure was formed after the PD/ZIF-8 nanoparticles were completely removed. We have previously reported that deposition of a thin layer of SWCNTs film on traditional MF membranes greatly improves the quality of the obtained PA active layer thanks to the high porosity, smoothness, and narrowly distributed pores of the SWCNT-coated support layer [28] . 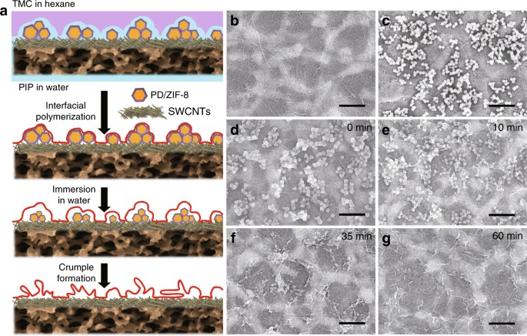Fig. 1 Evolution process of PA NF membrane with crumpled structures.aA schematic illustration showing the preparation process of nanoparticles-induced crumpled PA NF membrane. Top-view SEM images ofbpristine SWCNTs/PES composite membrane,cPD/ZIF-8 nanoparticles loaded SWCNTs/PES composite membrane.d–gMorphology change of the membrane immersed into water in different time after interfacial polymerization reaction on PD/ZIF-8 nanoparticles loaded SWCNTs/PES composite membrane (The scale bar of images is 1 μm). The PD/ZIF-8 nanoparticles loading mass is 4.3 μg cm−2. (TMC trimesoyl chloride, PIP piperazine, SWCNTs single-wall carbon nanotubes, PD polydopamine) To enhance the quality of the PA active layer, every SWCNT was wrapped by a thin PD layer before forming the SWCNTs network film (see Supplementary Figure 1 ). The PD-wrapped SWCNTs film enhanced the surface hydrophilicity to promote homogeneous distribution of the monomer solution for more controlled release of monomers during interfacial reaction. As a result, an ultrathin and defect-free PA layer was obtained. 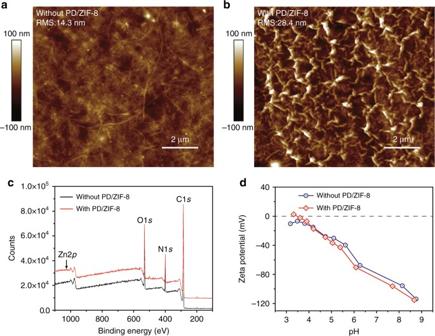Fig. 2 Morphology and chemical analysis of PA NF membranes.a,bAFM images (scale bar: 2 μm).cXPS survey spectra.dSurface zeta potential of PA NF membranes prepared from SWCNTs/PES composite membrane without PD/ZIF-8 nanoparticles loading and PD/ZIF-8 nanoparticles loaded SWCNTs/PES composite membrane. The PD/ZIF-8 nanoparticles loading mass is 4.3 μg cm−2 The thickness of PD/SWCNTs film used in this work was around 75 nm as confirmed by atomic force microscope (AFM) measurement (see Supplementary Figure 2a and 2b ). The SWCNTs film shows a uniform network structure with the effective pore size ranging from 10 to 20 nm (see Supplementary Figure 2c ). The surface chemical components of the SWCNTs film as analyzed by XPS confirms the existence of PD on carbon nanotubes (see Supplementary Figure 2d and 2e ). This PD layer renders the SWCNTs film hydrophilic as confirmed by a water contact angle (CA) of 22°. The evolution of the crumpled active layer of the TFC NF membrane was revealed by monitoring the change of membrane surface morphology at different stages during membrane fabrication process. The SEM image of the pristine SWCNTs film, covering the PES MF membrane before interfacial polymerization, suggests a smooth and transparent network structure formed by interconnected SWCNTs on the surface of PES MF membrane (Fig. 1b ). PD/ZIF-8 nanoparticles with an average diameter of ~150 nm were then loaded on this composite membrane to serve as the support layer as shown in Fig. 1c . The loading mass of PD/ZIF-8 nanoparticles on SWCNTs/PES composite membrane was 4.3 μg cm −2 . 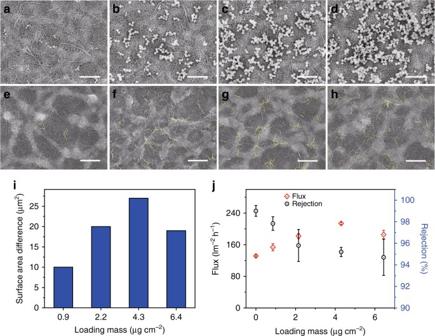Fig. 3 Influence of PD/ZIF-8 nanoparticles loading mass on crumple structure and membrane performance. SEM images of (a–d) PD/ZIF-8 nanoparticles loaded SWCNTs/PES composite membrane (scale bar: 1 μm) and (e–h) corresponding PA NF membranes with different PD/ZIF-8 nanoparticles loading mass (scale bar: 1 μm): (a,e) 0.9 μg cm−2; (b,f) 2.2 μg cm−2; (c,g) 4.3 μg cm−2, and (d,h) 6.4 μg cm−2.iSurface area difference between PA NF membranes prepared from SWCNTs/PES composite membrane with and without PD/ZIF-8 nanoparticles loading as a function of different loading mass.jFlux and rejection of PA NF membranes prepared with different PD/ZIF-8 nanoparticles loading mass. (Na2SO4concentration: 1000 ppm; applied pressure: 4 bar) The pristine ZIF-8 nanoparticles have smooth and sharp boundaries, whereas the PD/ZIF-8 nanoparticles, which are slightly larger, have rough and irregular boundaries due to the presence of the amorphous PD layer (see Supplementary Figure 3 ). The XRD spectroscopy reveals that the crystal structure of the ZIF-8 nanoparticles was unaffected by the PD coating (see Supplementary Figure 3 ). The thin PD coating was applied to improve the wetting property of ZIF-8 nanoparticles, which was confirmed by comparing the water CAs of different surfaces before and after modifications. 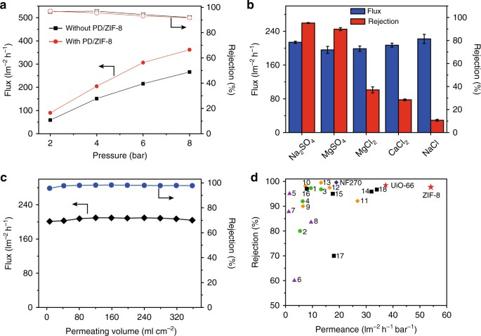Fig. 4 Desalination performance of PA NF membranes.aFlux and rejection of the PA NF membranes prepared from the SWCNTs/PES composite membrane with and without PD/ZIF-8 nanoparticles loading with respect to applied pressure (Na2SO4concentration: 1000 ppm).bVariation of flux and rejection of PA NF membranes prepared from PD/ZIF-8 nanoparticles loaded SWCNTs/PES composite membrane with respect to different salt solutions (salt concentration: 1000 ppm; applied pressure: 4 bar).cVariation of flux and rejection of PA NF membrane prepared from PD/ZIF-8 nanoparticles loaded SWCNTs/PES composite membrane as a function of permeating volume (Na2SO4concentration: 1000 ppm; applied pressure: 4 bar).dSummary of the filtration performance of the state-of-the-art NF membranes reported in literature in consideration of permeance and rejection for Na2SO4 Specifically, the CAs of the SWCNTs/PES composite membrane loaded with uncoated ZIF-8 nanoparticles and the SWCNTs/PES composite membrane loaded with PD/ZIF-8 nanoparticles were 53° and 36°, respectively (see Supplementary Figure 4 ). This result confirms that the PD layer effectively enhances the hydrophilicity of ZIF-8 nanoparticle. The improved hydrophilicity of the support layer could enhance interfacial polymerization reaction and consequently the quality of the PA layer (see Supplementary Figure 5 , Supplementary Figure 6 and Supplementary Table 1 ). After interfacial polymerization on the PD/ZIF-8 nanoparticles loaded SWCNTs/PES composite membrane, the membrane was immersed into water to release the ZIF-8 nanoparticles. Figure 1d–g are SEM images of the membrane with different immersion time. Before immersed into water, the PD/ZIF-8 nanoparticles and SWCNTs film could be clearly observed under the PA layer, indicating the top PA layer was rather thin and transparent (Fig. 1d ). The morphology of the PD/ZIF-8 nanoparticle was similar before and after interfacial polymerization reaction, which suggests that the PD/ZIF-8 nanoparticles were stable during the polymerization reaction (see Supplementary Figure 7 ). Immersion the membrane into water after polymerization promotes the gradual dissolution of the PD/ZIF-8 nanoparticles (Fig. 1e–g ). As the dissolution process continued, the crumpled surface morphology started to emerge and became growingly prominent until the PD/ZIF-8 nanoparticles dissolved completely (Fig. 1g ). The dissolution of ZIF-8 nanoparticles is ascribed to their instability in water at a low mass ratio of ZIF-8 to water [31] , [32] . A series of experiments were done to confirm such a dissolution mechanism. PD/ZIF-8 nanoparticles loaded SWCNTs/PES composite membranes were immersed into pure water, water containing 1 M Hmim and alkaline solution (pH: 13), respectively, for different time to observe whether the loaded PD/ZIF-8 nanoparticles dissolve or not. As shown in Supplementary Figure 8 , the PD/ZIF-8 nanoparticles were quickly dissolved and totally disappeared after 10 min when immersed the membrane in water. However, the PD/ZIF-8 nanoparticles could not dissolve at all in 1 M Hmim and alkaline solution even for a long immersing time up to 5 h (see Supplementary Figure 9 ). When the PD/ZIF-8 nanoparticles loaded SWCNTs/PES composite membrane after interfacial polymerization was immersed in 1 M Hmim solution, no PD/ZIF-8 nanoparticles were dissolved (see Supplementary Figure 10 ). This is because the existence of either Hmim ligand or OH − in the immersion solution could effectively suppress the hydrolysis of ZIF-8. In addition, the surface morphology of the NF membrane prepared from the SWCNTs/PES composite membranes without nanoparticles and with residual PD on the surface were also examined for comparison. No crumpled structure was observed in these cases (see Supplementary Figure 11-13 ), confirming that the formation of crumpled structure in the presence of PD/ZIF-8 nanoparticles was indeed induced by the PD/ZIF-8 nanoparticles. Fig. 1 Evolution process of PA NF membrane with crumpled structures. a A schematic illustration showing the preparation process of nanoparticles-induced crumpled PA NF membrane. Top-view SEM images of b pristine SWCNTs/PES composite membrane, c PD/ZIF-8 nanoparticles loaded SWCNTs/PES composite membrane. d – g Morphology change of the membrane immersed into water in different time after interfacial polymerization reaction on PD/ZIF-8 nanoparticles loaded SWCNTs/PES composite membrane (The scale bar of images is 1 μm). The PD/ZIF-8 nanoparticles loading mass is 4.3 μg cm −2 . (TMC trimesoyl chloride, PIP piperazine, SWCNTs single-wall carbon nanotubes, PD polydopamine) Full size image AFM was also applied to further evaluate the effect of PD/ZIF-8 nanoparticles on the morphology of PA active layer. Because commercial PES membranes have relatively significant intrinsic larger-scale roughness that would eclipse the smaller-scale roughness of the active layer to be formed, commercial anodic aluminum oxide (AAO) membrane (average pore diameter: 0.2 μm) with a smooth surface, instead of the rough PES membrane, was used as the support layer for surface characterization using AFM. Following the same approach for fabricating the NF membrane with PES composite support, a thin SWCNTs film was deposited onto the AAO membrane as a composite support for interfacial polymerization. The AFM images of PA NF membranes prepared using this SWCNTs/AAO composite support without and with PD/ZIF-8 nanoparticles as the sacrificial template are shown in Fig. 2a, b , respectively. In the absence of PD/ZIF-8 nanoparticles, the PA NF membrane prepared using the SWCNTs/AAO composite membrane yields a relatively smooth surface with root mean square (RMS) roughness of 14.3 nm (Fig. 2a ), with the underlying SWCNTs film clearly observable through the active layer. In comparison, the PA NF membrane prepared using the SWCNTs/AAO composite membrane with PD/ZIF-8 nanoparticles forms a crumpled surface structure full of ridges, with an RMS roughness of 28.4 nm (Fig. 2b ). The thickness of crumpled PA layer was estimated by using focus ion beam-scanning electron microscope (FIB-SEM) technology (see Supplementary Figure 14 ). As shown in Supplementary Figure 14 , the thickness of PA active layer is around 8–14 nm. This value is similar to the thickness of PA layer prepared without PD/ZIF-8 nanoparticles as reported in our previous work [28] . The chemical composition of the PA active layers obtained thereby was analyzed by X-ray photoelectron spectroscopy (XPS). The XPS spectra of the two PA active layers, one formed with PD/ZIF-8 nanoparticles and the other without, suggest that they have the same chemical composition with equal abundance of C, N, and O (Fig. 2c ). No Zn element was detected (the Zn2 p peak is usually centered at 1044.8 eV) in these spectra, confirming that all ZIF-8 nanoparticles were removed and no residual remained in the final PA active layer. Based on the O/N elemental ratio from the XPS spectra, the degrees of crosslinking of the PA active layers were calculated [33] , [34] . The degrees of crosslinking of PA active layers prepared from SWCNTs/PES composite support without and with PD/ZIF-8 nanoparticles loading are 77.6% and 60.3%, respectively (Table 1 ), suggesting that the presence of PD/ZIF-8 nanoparticles reduces the degree of crosslinking of the PA active layer. It is worth to noting that the crosslinking degree is still high, which ensures the rejection performance of PA NF. In addition, the MWCO of PA NF membranes prepared with and without PD/ZIF-8 nanoparticles loading was measured to investigate the effect of crosslinking degree. Our results show that the MWCO for PA NF membrane without PD/ZIF-8 is 400 and the MWCO for PA NF membrane with PD/ZIF-8 is 410 (see Supplementary Figure 15 ). It indicates that the two membranes have similar MWCO. Fig. 2 Morphology and chemical analysis of PA NF membranes. a , b AFM images (scale bar: 2 μm). c XPS survey spectra. d Surface zeta potential of PA NF membranes prepared from SWCNTs/PES composite membrane without PD/ZIF-8 nanoparticles loading and PD/ZIF-8 nanoparticles loaded SWCNTs/PES composite membrane. The PD/ZIF-8 nanoparticles loading mass is 4.3 μg cm −2 Full size image Table 1 Surface chemical components of PA NF membranes prepared from SWCNTs/PES composite membrane with and without PD/ZIF-8 nanoparticles loading Full size table The C1 s , O1 s , and N1 s peaks of the XPS spectra (see Supplementary Figure 16 ), which provide more detailed information of the chemical compositions of PA active layer, are summarized in Table 1 . The fractions of carboxylic acid groups and unreacted amine groups in the PA active layer prepared with the PD/ZIF-8 nanoparticles loaded SWCNTs/PES composite support were 19.5% and 6.3%, respectively; whereas the corresponding fractions of the PA active layer prepared using SWCNTs/PES composite membrane without PD/ZIF-8 nanoparticles were 13.4% and 5.4%, respectively. We also measured the zeta potential of the PA active layers due to its significant impact on solute rejection. The results suggest that the presence of PD/ZIF-8 nanoparticles, which drastically affects the morphology of the PA active layer, does not seem to have significant impact on the zeta potential of the PA active layer. Both PA active layers are negatively charged to a similar extent when pH was above 3.5 (Fig. 2d ). The PA active layers acquire very strong negative zeta potentials at neutral and high pH, which is beneficial to the rejection of divalent or multivalent ions via the Donnan effect [35] , [36] , [37] . Effect of loading mass and size of nanoparticles on crumple structure The effect of loading mass and size of PD/ZIF-8 nanoparticles on the structure of PA active layer was also investigated in detail. Figure 3 a–d show the SEM images of PD/ZIF-8 nanoparticles loaded SWCNTs/PES composite support with the loading mass systematically increasing from 0.9 μg cm −2 to 6.4 μg cm −2 . The morphologies of the resulting PA active layers (Fig. 3 e–h) suggest that more crumpled structure resulted from higher loading mass of PD/ZIF-8 nanoparticles. Based on their AFM images, we also compared the surface area (i.e., actual area per projected area) of the PA active layers prepared with different loading mass of PD/ZIF-8 nanoparticles (see Supplementary Figure 17 ), using a built-in function of the AFM software that estimates the surface area based on the tortuous paths the AFM tip travels under tapping mode. While such an approach for area estimation has its limitations (e.g., it cannot measure area of the down-facing regions), it nonetheless provides useful information for a semi-quantitative comparison to elucidate the impact of PD/ZIF-8 loading on enhancing the PA active layer area. Here, we compare the area difference between the PD/ZIF-8 templated PA active layer and PA active layer prepared without PD/ZIF-8, and express this area difference as a function of mass loading of PD/ZIF-8 nanoparticles (Fig. 3i ). Such surface area differences for PA active layers with PD/ZIF-8 nanoparticles loading mass of 0.9 μg cm −2 , 2.2 μg cm −2 , and 4.3 μg cm −2 were 10 μm 2 , 20 μm 2 , and 27 μm 2 , respectively, suggesting that surface area increases with increasing PD/ZIF-8 nanoparticles loading mass. However, further increasing the loading mass to 6.4 μg cm −2 reduces the surface area difference to 19 μm 2 . NF experiments with 1000 ppm Na 2 SO 4 solution suggests that the change of membrane flux positively correlates with the change in surface area, with only a slight compromise in salt rejection as the surface area increases (Fig. 3j ). For example, with a PD/ZIF-8 mass loading of 4.3 μg cm −2 , the permeating flux reaches a maximum of 214 l m −2 h −1 , with the rejection of Na 2 SO 4 slightly reduced to ~95%. Interestingly, the measured percentage increase of permeance was more significant than the percentage increase of actual PA active layer area. One possible explanation is that the templated active layer has a weakened binding with the underlying support, which increases the fraction of highly permeable PA active layer compared to that prepared using a conventional non-templating approach. Hereafter, we chose to fix the PD/ZIF-8 nanoparticle mass loading at 4.3 μg cm −2 to prepare PA NF membranes for further comprehensive investigation, as such a loading yields the most permeable membrane with a satisfactory rejection. Fig. 3 Influence of PD/ZIF-8 nanoparticles loading mass on crumple structure and membrane performance. SEM images of ( a – d ) PD/ZIF-8 nanoparticles loaded SWCNTs/PES composite membrane (scale bar: 1 μm) and ( e – h ) corresponding PA NF membranes with different PD/ZIF-8 nanoparticles loading mass (scale bar: 1 μm): ( a , e ) 0.9 μg cm −2 ; ( b , f ) 2.2 μg cm −2 ; ( c , g ) 4.3 μg cm −2 , and ( d , h ) 6.4 μg cm −2 . i Surface area difference between PA NF membranes prepared from SWCNTs/PES composite membrane with and without PD/ZIF-8 nanoparticles loading as a function of different loading mass. j Flux and rejection of PA NF membranes prepared with different PD/ZIF-8 nanoparticles loading mass. (Na 2 SO 4 concentration: 1000 ppm; applied pressure: 4 bar) Full size image ZIF-8 nanoparticles with other sizes, ∼ 30 nm, ∼ 100 nm, ∼ 200 nm, and ∼ 400 nm were also used to fabricate PA NF membrane with same loading mass as ZIF-8 nanoparticles of ∼ 150 nm (see Supplementary Figure 18 and Supplementary Table 2 ). These PD/ZIF-8 nanoparticles were loaded onto SWCNTs/PES composite membranes for interfacial polymerization, respectively. Supplementary Figure 19 shows that all PD/ZIF-8 nanoparticles were successfully dissolved and crumpled PA layer were achieved especially when the ZIF-8 nanoparticles larger than 30 nm. With the increase of PD/ZIF-8 nanoparticle size, larger crumple structures were generated. The desalination performance of the corresponding PA NF membranes were tested (see Supplementary Figure 20 ). The permeating fluxes are 213, 200, and 214 l m −2 h −1 corresponding to the ZIF-8 nanoparticle size of 30, 100, and 150 nm, respectively. Meanwhile, the corresponding rejections to Na 2 SO 4 are 95, 96, and 95.3%, respectively. Further increasing the nanoparticles size to 200 nm and 400 nm, the corresponding permeating flux decreases to 157 and 171 l m −2 h −1 with rejection of 92% and 95.7%, respectively. Desalination performance of PA NF membranes The impacts of applied pressure on the permeate flux and salt rejection were also investigated using 1000 ppm Na 2 SO 4 for both PA NF membranes with and without PD/ZIF-8 nanoparticles templating. For both membranes, the permeating fluxes increase proportionally with increasing applied pressure at low pressure range, but level off at higher pressure range due to concentration polarization (Fig. 4a ) [36] , [38] . The PA NF membrane templated with PD/ZIF-8 nanoparticles exhibits higher fluxes than the membrane without PD/ZIF-8 nanoparticles templating throughout the whole pressure range, while they exhibit similar rejection rate to Na 2 SO 4 . With increasing applied pressure, the rejection rates for both membranes decrease slightly from 97% at 2 bar to 92% at 6 bar. For the PA NF membrane prepared without PD/ZIF-8 template, the rejection rate was relatively independent of Na 2 SO 4 feed concentration, remaining ~97% as the feed concentration increased from 1000 ppm to 6000 ppm. For PA NF membrane prepared with PD/ZIF-8 nanoparticles loading, the rejection rate decreased slightly from ~97% at 1000 ppm to ~94% at 6000 ppm (see Supplementary Figure 21 ). Filtration performance of our PA NF membrane with other salts was also evaluated (Fig. 4b ). While the templated PA NF membrane exhibit similar permeating fluxes with all salts tested, the salt rejections for Na 2 SO 4 and MgSO 4 are much higher than for MgCl 2 , CaCl 2 , and NaCl possibly due to the synergistic effect of strong Donnan exclusion and size sieving with the sulfate salts. The performance of the templated PA NF membrane is also stable over time. In experiments with 1000 ppm Na 2 SO 4 feed solution and an applied pressure of 4 bar, no appreciable change of permeating flux and salt rejection was observed in continuous filtration up to a permeate volume per area of 360 ml cm −2 (Fig. 4c ). Fig. 4 Desalination performance of PA NF membranes. a Flux and rejection of the PA NF membranes prepared from the SWCNTs/PES composite membrane with and without PD/ZIF-8 nanoparticles loading with respect to applied pressure (Na 2 SO 4 concentration: 1000 ppm). b Variation of flux and rejection of PA NF membranes prepared from PD/ZIF-8 nanoparticles loaded SWCNTs/PES composite membrane with respect to different salt solutions (salt concentration: 1000 ppm; applied pressure: 4 bar). c Variation of flux and rejection of PA NF membrane prepared from PD/ZIF-8 nanoparticles loaded SWCNTs/PES composite membrane as a function of permeating volume (Na 2 SO 4 concentration: 1000 ppm; applied pressure: 4 bar). d Summary of the filtration performance of the state-of-the-art NF membranes reported in literature in consideration of permeance and rejection for Na 2 SO 4 Full size image The NF performance in terms of permeance and salt rejection of our PD/ZIF-8 templated PA NF membrane is compared with the performance of the state-of-the-art NF membranes reported in literatures [14] , [28] , [29] , [30] , [39] , [40] , [41] , [42] , [43] , [44] , [45] , [46] , [47] , [48] , [49] , [50] , [51] , [52] , [53] , [54] , [55] (Fig. 4d , Supplementary Figure 22 and Supplementary Ref. 1 - 21 ). The comparison suggests that the performance of templated PA NF membrane is, to a large extent, superior to all other membranes recently developed by others including thin film nanocomposite membranes [39] , [40] , [41] , [42] (marked as green circle of 1–4 in Fig. 4d , see also Supplementary Ref. 1 - 4 ), 2D nanomaterials-assembled membranes [43] , [44] , [45] , [46] (marked as purple triangle of 5–8 in Fig. 4d , see Supplementary Ref. 5 - 8 ), PA NF membranes prepared with various monomers [47] , [48] , [49] , [50] , [51] (marked as orange rhombus of 9–13 in Fig. 4d , see Supplementary Ref. 9 - 13 ), membranes prepared with modification of support layers [28] , [29] , [30] , [52] , [53] (marked as black square of 14–18 in Fig. 4d , see Supplementary Ref. 14 - 18 ), and commercial NF membrane (e.g., NF270 by Dow). The templated PA NF membrane shows several folds of increase in permeance compared to most other NF membranes, while maintaining a high salt rejection simultaneously. It is worth noting that a large applied pressure around 6 to 8 bar is usually required to operate with common NF membranes. However, the templated PA NF membrane developed in this work could be operated with a much lower applied pressure, e.g., generating a permeating flux of 90 l m −2 h −1 with only 2 bar. To further demonstrate the role of PD/ZIF-8 nanoparticles as sacrificial template, a control experiment was done where water-stable UiO-66 MOF nanoparticles was synthesized and loaded onto the SWCNTs/PES composite membrane to fabricate PA NF membrane (see Supplementary Figure 23 and 24 ). Our results show that the introduction of PD/UiO-66 nanoparticles on the SWCNTs/PES composite membrane could improve the flux of the resulting PA NF membrane also at a certain extent (see Supplementary Figure 25 ). A maximum permeance of 36.7 l m −2 h −1 bar −1 meanwhile a rejection of ~97% for Na 2 SO 4 at the nanoparticles loading mass of 8.6 μg cm −2 was achieved (marked as UiO-66 in Fig. 4d ). This permeance is slightly higher than the PA NF membrane prepared from SWCNTs/PES composite membrane without nanoparticles loading, but still much lower than that of PA NF membrane prepared from PD/ZIF-8 nanoparticles. It confirms that the crumple structure is beneficial to the increase of available area for water permeation. We described above the use of ZIF-8 nanoparticle as sacrificial template to induce the formation of crumpled structure on PA NF membrane. The results reveal that the geometric structure of ZIF-8 nanoparticles provides a rough surface structure on support layer and dominates the formation of the crumpled structure. From this point of view, other kinds of nanoparticles those can be easily removed by mild post-treatment can also be used as sacrificial template instead of ZIF-8 nanoparticle. Here, ZIF-67 nanoparticles (300–500 nm in diameter) and calcium carbonate (CaCO 3 ) nanoparticles ( ∼ 100 nm in diameter) were chosen as sacrificial nanomaterials. Our results show that the crumpled PA layers could also be obtained as shown in Supplementary Figure 26 and 27. The permeating flux of the two membranes are 183 l m −2 h −1 for PD/ZIF-67 nanoparticles loading and 191 l m −2 h −1 for PD/CaCO 3 nanoparticles loading, with Na 2 SO 4 rejection of 97.2 and 96.5%, respectively (see Supplementary Table 3 ). These values are still much higher than that of the membrane without nanoparticles loading. These results indicate that other soluble nanoparticles could also be used as sacrificial template to play the same role as ZIF-8 nanoparticles. Overall, we have developed a strategy to design sacrificial nanoparticles templated PA NF membranes with unprecedentedly high permeance and a satisfactorily high rejection for desalination. The nanoparticles, preloaded to the SWCNTs/PES support, acted as a sacrificial template to create a PA active layer with extensive crumpled surface morphology, which consequently yielded a higher specific surface area and a larger fraction of highly permeable PA skin layer. The morphology of the crumpled surface and the surface area of PA active layer can be fine-tuned by controlling the loading mass and particle size of sacrificial nanoparticles. As a result, an ultrahigh permeance, up to 53.5 l m −2 h −1 bar −1 , together with a reasonably high rejection of 95.3% was achieved for a feed solution of 1000 ppm Na 2 SO 4 when PD/ZIF-8 was used as sacrificial template. This work provides a strategy to design TFC membrane with extremely high permeance that is radically different from those by modifying the molecular structure of the active layer, which could only achieve a higher permeance at the cost of comprising rejection. An NF membrane with ultrahigh permeance and reasonably high salt rejection is very promising for more energetically and kinetically efficient treatment of low-salinity water, which has great potential in advancing brackish groundwater desalination, water softening, household RO/NF, and wastewater reuse. In consideration of the easy and scalable synthesis process of various nanoparticles, the use of them as sacrificial nanomaterials should be feasible for scaling up the resulting PA NF membranes. From the practical application viewpoint, one of the main issue is to develop more effective technology for nanoparticle loading to replace the present filtration based deposition process. General Materials used in this work and detailed synthesis of PD decorated nanoparticles, such as PD/ZIF-8, PD/ZIF-67, PD/CaCO 3 , and PD/UiO-66, have been shown as Materials and Synthesis in Supplementary methods. Preparation of SWCNTs/PES composite membrane PD/SWCNTs dispersion was prepared as follows: 20 mg SWCNT and 200 mg sodium dodecyl benzene sulfonate was added into 200 ml deionized water and sonicated for 36 h by using ultrasonic cleaning machine with 300 W power. The SWCNT dispersion was then centrifuged for 30 min at 10,000 rpm and 150 ml supernatant was collected. The 150 ml supernatant was diluted into 300 ml by using pure water and 30 mg dopamine was then added into it. After stirring for 1 h at 40 °C, 30 ml 0.1 mol l −1 Tris buffer (pH 8.5) was added into the system to further react for 36 h at 40 °C. The obtained PD/SWCNT dispersion was centrifuged for 30 min at 10,000 rpm, the supernatant was collected and preserved at 4 °C. The SWCNTs/PES composite membrane was prepared by depositing the PD/SWCNTs onto PES microfiltration membrane via vacuum filtration process according to our previously report [56] , [57] . Specifically in this work, a certain amount of collected PD/SWCNTs supernatant was diluted by 40 times with ethanol and vacuum-filtrated onto PES microfiltration membrane at 0.02 MPa vacuum pressure. The resulting density of PD/SWCNTs on PES microfiltration membrane is 5 μg cm −2 . Preparation of nanoparticles loaded SWCNTs/PES composite membrane PD/ZIF-8 nanoparticles loaded SWCNTs/PES composite membrane was prepared as follows: Taking 4.3 μg cm −2 loading mass as an example, 1 ml 0.05 mg ml −1 PD/ZIF-8 nanoparticles dispersion was diluted to 50 ml with ethanol and then deposited onto a 11.6 cm 2 SWCNTs/PES composite membrane via vacuum filtration at 0.02 MPa. After dried at 60 °C for 2 min, PD/ZIF-8 nanoparticles loaded SWCNTs/PES composite membrane was obtained. PD/UiO-66 nanoparticles loaded SWCNTs/PES composite membrane, PD/ZIF-67 nanoparticles loaded SWCNTs/PES composite membrane, and PD/CaCO 3 nanoparticles loaded SWCNTs/PES composite membrane were all prepared in the same procedure as PD/ZIF-8 nanoparticles loaded SWCNTs/PES composite membrane with same loading mass. As for the PD/ZIF-8 nanoparticles loaded SWCNTs/PES composite membranes with different PD/ZIF-8 nanoparticles loading mass, different volumes of 0.05 mg ml −1 PD/ZIF-8 nanoparticles dispersion were used: 0.21 ml for achieving 0.9 μg cm −2 , 0.51 ml for achieving 2.2 μg cm −2 , and 1.49 ml for achieving 6.4 μg cm −2 . Interfacial polymerization Interfacial polymerization was conducted at 25 °C and relative humidity of about 60%. In a typical procedure, a piece of nanoparticles loaded SWCNTs/PES composite membrane was put onto a glass plate where a few drops of PIP aqueous solution ( ∼ 0.5 ml) was preloaded. An aliquot of 2 ml aqueous solution containing 2.5 mg ml −1 PIP and 0.75 mg ml −1 polyvinyl pyrrolidone (K-30) was dropped onto the membrane and stood for 30 s. The excess PIP solution was removed by drained glass plate vertically in air until no obvious water spot can be observed on the membrane. An aliquot of 2 ml hexane containing 2 mg ml −1 TMC was then dropped onto the above wetted membrane where the edge of the membrane was sealed by a filter cup and stood for 30 s. After removing the excess TMC solution, the membrane was immersed into hexane for 30 s to remove unreacted TMC and then oven-cured at 60 °C for 30 min to obtain PA NF membrane. In order to remove nanoparticles, the obtained PA NF membrane was immersed in water in a prescribed time and then washed by water for three to five times. The resulting membrane was stored in water at 4 °C for use. Characterization SEM images were taken from a Hitachi S4800 cold field-emission scanning electron microscopy. TEM images were acquired from a FEI Tecnai G2 F20 S-TWIN 200KV field-emission transmission electron microscopy. AFM images were obtained in tapping mode of a Bruker Dimension Icon atomic force microscopy. XRD was tested by a Bruker AXS D8 Advance powder X-Ray diffractomer. Surface Zeta potential was tested on an Anton Paar Surpass solid surface analysis. Water CA was measured on a Data-Physics OCA 20 with 2 μl water droplet. XPS was taken from a Thermo Fisher Scientific ESCALAB 250Xi X-Ray photoelectron spectrometer. Total organic carbon (TOC) was detected by OI Analytical Aurora Model 1030. FIB-SEM images were obtained from a FEI field-emission type scanning electron microscope equipped with focus ions beam device (Scios). The effective membrane pore size of membranes were determined by filtration of a group of polyethylene glycol (PEG) molecules with different molecular weights (200, 400, 600, and 1000 Da, respectively) [58] . An aliquot of 200 ppm PEG aqueous solutions were used as feed solutions to permeate the membrane at applied pressure of 4 bar. Rejection was calculated from the contents of TOC of feed and filtrate solutions, respectively, as obtained by a TOC Analyzer. MWCO was obtained according to the molecular weight where the rejection is 90%. Stokes radius of PEG can be calculated according to its average molecular weight based on the following equation (Eq. 1 ): 
    r_p = 16.73×10^ - 12× M^0.557
 (1) where M is molecular weight of solutes, and r p is the Stokes radius. Membrane performance test A cross-flow NF apparatus with a separation area of 7.1 cm 2 was used to test the membrane performance at room temperature. Rejection was calculated from conductivity of feed and filtrate solutions using Eq. ( 2 ), where C f and C p represent conductivity of feed solution and permeate, respectively. R = (1 - C_p/C_f)×100%
 (2) Flux J is determined by Eq. ( 3 ), where Δ w is weight increase of permeate during filtration time Δ t , A is the separation area of the cell, ρ is density of permeate and we here consider it to be 1 g ml −1 because its low salt concentration. J = Δ w/ρ AΔ t
 (3) Here, Permeance is defined as flux per unit applied pressure, see in Eq ( 4 ), where Δ P is the applied transmembrane pressure for filtration experiment. Permeance = J/Δ P
 (4) Data availability The authors declare that all of the data supporting the finding of this study are available within the paper and supplementary information and also are available from the corresponding author upon reasonable request.